High-throughput hyperdimensional vertebrate phenotyping Most gene mutations and biologically active molecules cause complex responses in animals that cannot be predicted by cell culture models. Yet animal studies remain too slow and their analyses are often limited to only a few readouts. Here we demonstrate high-throughput optical projection tomography with micrometre resolution and hyperdimensional screening of entire vertebrates in tens of seconds using a simple fluidic system. Hundreds of independent morphological features and complex phenotypes are automatically captured in three dimensions with unprecedented speed and detail in semitransparent zebrafish larvae. By clustering quantitative phenotypic signatures, we can detect and classify even subtle alterations in many biological processes simultaneously. We term our approach hyperdimensional in vivo phenotyping. To illustrate the power of hyperdimensional in vivo phenotyping, we have analysed the effects of several classes of teratogens on cartilage formation using 200 independent morphological measurements, and identified similarities and differences that correlate well with their known mechanisms of actions in mammals. Large-scale screening of phenotypes induced by small molecules, natural products, gene mutations and other agents is essential for all fields of modern biology and drug discovery. Although cell-based assays are amenable to high-throughput screening (HTS), results often fail to translate to animal models and clinical trials. Even the most sophisticated in vitro models fail to preserve the complexity and architecture of intact organs and in vivo processes such as disease pathology, tissue homoeostasis and drug-induced toxicity. To address these limitations, chemical screens are increasingly being conducted using zebrafish ( Danio rerio ) [1] , a small vertebrate model organism that is widely used for genetic screens and amenable to high-throughput methodologies. To date, however, chemical screens in zebrafish have typically ignored phenotypes not encompassed by more than a small number of predefined readouts. The most ambitious efforts have focused on behavioural phenotypes and simultaneously assessed up to a few dozen readouts [2] , [3] . Similarly, although large-scale genetic screens have been carried out for decades in zebrafish, the readouts are often non-quantitative and limited to easily observed features. Morphological phenotyping remains a subjective process that can vary greatly between locales and lacks the systematization and throughput required for HTS. To fully realize the potential of genetic and small molecule screens in vertebrates, it will be necessary to adopt a phenomics approach in which hundreds of morphological parameters are quantified and interpreted using unbiased, automated techniques similar to those developed for high-content screening (HCS) of cells. For this purpose, we demonstrate a high-throughput optical projection tomography (OPT) system that can generate three-dimensional (3D) images of entire zebrafish larvae at micrometre resolution within tens of seconds per larva (including all animal handling steps), an order of magnitude faster than existing OPT systems. Our system uses simple fluidics and image processing algorithms, and can be readily adapted to a variety of standard microscopes to rapidly generate micrometre-resolution 3D reconstructions of entire organs or other complex morphological features that have been labelled with standard histological dyes or by whole-mount in situ hybridization (WISH) or immunohistochemistry. This technique allows us to rapidly profile complex phenotypes in an unbiased manner using hundreds of independent morphological measurements on large numbers of animals. By hierarchically clustering the phenotypic signatures obtained under multiple screened conditions, we are then able to identify chemicals that act through related or different pathways in vivo . We term our approach hyperdimensional in vivo phenotyping (HIP). High-throughput OPT High-content in vivo phenotyping of vertebrate model organisms necessitates rapid 3D imaging of large volumes of tissue. Conventional 3D imaging techniques, such as confocal and two-photon microscopy, rely on optically sectioning the specimen and are too slow for HTS of phenotypes that encompass large regions of the body. Selective plane illumination microscopy [4] , [5] offers increased throughput, but suffers in samples containing opaque or highly scattering regions and is poorly suited for imaging larvae with developed organs. All of these techniques are dependent on fluorescent signals and cannot be adapted for commonly used chromogenic stains. OPT [6] is a 3D imaging technique that computationally obtains volumetric information from collections of 2D images acquired at multiple sample angles. OPT is less subject to interference from intervening regions, has sufficient penetration depth to image an entire zebrafish larvae, and is compatible with both coloured dyes and fluorescent reporters [6] , [7] . In addition, unlike confocal and other optical slicing techniques, OPT yields rotationally symmetric voxels and therefore provides rotationally unbiased measurements. However, the throughputs of existing OPT systems are severely limited (acquisition times of 5–30 min per specimen) due to the complexity involved in sample preparation. The need to embed samples in agar or similar materials to stabilize them for precision rotation and image acquisition renders large-scale screens unfeasible [6] , [8] . To avoid this limitation, we have developed a high-throughput OPT system that can handle and image entire non-embedded animals at micrometre resolution in tens of seconds by automatically correcting for errors due to animal movement and other artifacts ( Fig. 1 ). 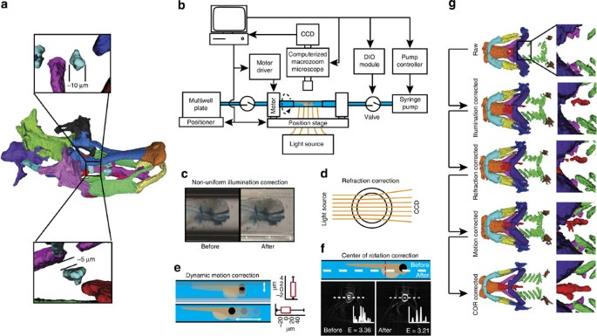Figure 1: High-throughput optical projection tomography. (a) Tomographic reconstruction of the craniofacial cartilage after image processing. Insets show details of the hypobranchial bone. The resolution of the 3D reconstruction is sufficient to distinguish bones with dimensions of ~10 μm and gaps of ~5 μm between bones. (b) Schematic representation of the OPT platform. A fluidic system composed of a pump, valves and tubing is used to load larvae from multiwell plates into a glass capillary located within the field-of-view of a macrozoom microscope. The capillary is held at two ends by stepper motors with hollow shafts that sit on a position stage. Several dynamic image artifact correction steps are performed before reconstruction. (c) Non-uniformity of illumination due to the capillary walls is corrected. (d) The light path through the capillary is simulated and is fed to the reconstruction algorithm to correct for the refraction of light by the capillary. (e) Small movements of the larva along the capillary axis and radial vibrations of the capillary are detected and corrected. The box-plots quantify the vibrations of the capillary (top plot) and the motion of the larva along the capillary axis (bottom plot) before correction. (f) Identification of centre of rotation (COR) for reconstruction. Reconstructing a cross-section using different COR estimates allows us to identify the true rotation axis with micrometre precision. The bottom panels show reconstructions using two different CORs. The reconstruction on the left corresponds to a COR estimated solely from the boundaries of the capillary sidewalls. The reconstruction on the right has sharper boundaries and lower entropy, and is therefore selected as the best estimate for true COR. Graphs show 1D intensity profiles across the dashed lines. Entropy of each image is shown on the bottom right corner. (g) Each step of image artifact correction produces increasingly accurate tomographic reconstructions. Images show 3D reconstructions from 320 images of a 5-dpf zebrafish larvae stained with Alcian blue. Insets show zoomed views of the most posterior region of the basihyal cartilage (red). Figure 1: High-throughput optical projection tomography. ( a ) Tomographic reconstruction of the craniofacial cartilage after image processing. Insets show details of the hypobranchial bone. The resolution of the 3D reconstruction is sufficient to distinguish bones with dimensions of ~10 μm and gaps of ~5 μm between bones. ( b ) Schematic representation of the OPT platform. A fluidic system composed of a pump, valves and tubing is used to load larvae from multiwell plates into a glass capillary located within the field-of-view of a macrozoom microscope. The capillary is held at two ends by stepper motors with hollow shafts that sit on a position stage. Several dynamic image artifact correction steps are performed before reconstruction. ( c ) Non-uniformity of illumination due to the capillary walls is corrected. ( d ) The light path through the capillary is simulated and is fed to the reconstruction algorithm to correct for the refraction of light by the capillary. ( e ) Small movements of the larva along the capillary axis and radial vibrations of the capillary are detected and corrected. The box-plots quantify the vibrations of the capillary (top plot) and the motion of the larva along the capillary axis (bottom plot) before correction. ( f ) Identification of centre of rotation (COR) for reconstruction. Reconstructing a cross-section using different COR estimates allows us to identify the true rotation axis with micrometre precision. The bottom panels show reconstructions using two different CORs. The reconstruction on the left corresponds to a COR estimated solely from the boundaries of the capillary sidewalls. The reconstruction on the right has sharper boundaries and lower entropy, and is therefore selected as the best estimate for true COR. Graphs show 1D intensity profiles across the dashed lines. Entropy of each image is shown on the bottom right corner. ( g ) Each step of image artifact correction produces increasingly accurate tomographic reconstructions. Images show 3D reconstructions from 320 images of a 5-dpf zebrafish larvae stained with Alcian blue. Insets show zoomed views of the most posterior region of the basihyal cartilage (red). Full size image The system is simple and comprised a standard computerized syringe pump and fluidic components ( Fig. 1b ) that automatically loads individual zebrafish into a fluid-filled ultrathin borosilicate glass capillary, which we have recently shown to provide excellent imaging characteristics [9] . The capillary is held by two stepper motors that rotate the capillary through its main axis. With this system we are able to handle, rotate and image from multiple angles entire larvae [9] , [10] . Unlike previous techniques, our method does not require larvae to be embedded, thereby eliminating the slowest and most labour-intensive step in OPT imaging. Live or fixed larvae are first automatically positioned in the capillary. Larvae are then rapidly rotated through 360°, allowing images to be continuously acquired at a high frame rate from multiple angles. However, OPT reconstruction of such non-embedded samples present several new challenges that we first needed to address. Tomography algorithms require that the sample remains stationary and evenly illuminated during image acquisition. Additionally, the centre of rotation (COR) of the imaged sample must be precisely known. Therefore, non-embedded samples need to be analysed for (i) non-uniform illumination of the capillary ( Fig. 1c ), (ii) refraction of light by the glass walls of the capillary ( Fig. 1d ), (iii) motion artifacts arising from vibrations of the capillary and fluctuations in the fluidic pressure along the capillary ( Fig. 1e ) and (iv) precise determination of the sample’s COR ( Fig. 1f ). We have developed algorithms that allow us to dynamically correct for each of these artifacts in every image frame. Before the image correction steps, an algorithm first determines the larva’s orientation (head-first or tail-first) within the capillary [9] and then aligns the capillary along the horizontal axis in each image by identifying its sidewalls through a Hough transformation. Next, an algorithm corrects for non-uniform illumination between the sidewalls and the central axis of the capillary by first calculating average pixel intensities across regions containing no larva, which are then used as a baseline to equalize illumination in all regions of the capillary ( Fig. 1c ). Two different types of motion artifacts arise during the imaging of non-embedded samples: vibration of the capillary and longitudinal movement of the larvae within the capillary due to fluctuations in the fluidic pressure. Vibrations are automatically compensated for by identifying the sidewalls of the capillary. These landmarks are used to align all the images acquired at different angles and to stretch or shrink the images to equalize the capillary diameters across images. Longitudinal motions are automatically compensated for by identifying a prominent anterior feature (for example, the tip of the head) and using this as a reference point to precisely align the larva across all the images ( Fig. 1e and Supplementary Fig. S1 ). Estimating the COR by simply calculating the midpoint between the sidewalls of the capillary is insufficient for high-resolution reconstructions ( Fig. 1f ‘Before’). We therefore automatically refine the COR estimate by using a filtered back-projection algorithm to compute multiple reconstructions of a single 2D transverse slice through the larva under different estimated CORs deviating slightly from the initial estimate. The COR whose reconstruction has the sharpest boundaries (that is, lowest entropy) is considered to be the true COR and is used for the subsequent 3D reconstruction of the entire larva ( Fig. 1f ‘After’ and Supplementary Fig. S2 ). The corrected images are reconstructed using an order-subset expectation-maximization (OSEM) algorithm. To produce the most accurate 3D reconstruction possible, the algorithm must take into account the refraction of light as it passes through the walls of the borosilicate glass capillary. To do this, we have modelled the path followed by parallel light rays originating from a source below the capillary and propagated them back to a virtual imaging plane ( Fig.1d and Supplementary Fig. S3 ). Using these algorithms, we can produce 3D reconstructions of non-embedded zebrafish larvae with micrometre resolution ( Fig. 1a and g ). For example, we are able to reliably detect individual bones and features of the segmented craniofacial skeleton (described below) with dimensions smaller than 10 μm and distinguish these from other structures located within only 5 μm. The overall throughput for all imaging and handling steps is 18 s per larva (see Supplementary Table S1 ). All steps of the OPT imaging process are automated, including the loading and positioning of the larva, capillary rotation, multi-angle image acquisition, unloading of larva and movement of the loading nozzle to the subsequent well. During standard operation, the image acquisition rate is primarily governed by the camera’s frame rate and the number of images acquired at different angles of rotation. To minimize the acquisition time we employ a high-speed CCD (Charge-coupled-device) camera capable of acquiring 128 frames per second. We find that 320 images acquired as the sample is rotated through 360° are sufficient for accurate, high-resolution tomographic reconstruction. This allows a single larva to be imaged within only 2.5 s (that is, exposure time of ~8 milliseconds). 3D image reconstruction from acquired multi-angle images is done automatically and offline; therefore it does not limit the speed of data acquisition and screening. Using a basic computer with a single processor, a 3D image with 250 × 250 × 450 pixels takes 3.5 min to reconstruct with the OSEM algorithm. For large-scale screens, image reconstruction can be easily accelerated by using multi-core computers or computer clusters. Assessment of craniofacial abnormalities Histological dyes and chromogenic substrates (for example, Alcian blue, NBT/BCIP) modify the colour or opaqueness of samples and are commonly used to label specific tissues. 3D reconstructions from samples labelled with these stains maintain their colour properties, allowing features of interest to be computationally extracted through image analysis. The craniofacial skeleton stained with Alcian blue is particularly attractive for 3D analysis due to its high level of organizational complexity. To analyze craniofacial cartilage, we employ a colour-based linear discriminator model based on previous training data to automatically identify voxels associated with stained tissue based on their RGB values. Using this approach, we are able to successfully separate the craniofacial skeleton from surrounding tissues with exquisite precision and accuracy ( Fig. 1a ). The isolated craniofacial skeleton is subsequently segmented into individual bones using a semiautomated but rapid algorithm. Using segmented 3D reconstructions from our system, we can visualize individual craniofacial bones and substructures with dimensions smaller than 5 μm ( Fig. 1a ). The voxel size used for the craniofacial assessment described below is 2.25 × 2.25 × 2.25 μm, which is sufficient to accurately assess the morphology of all bones in zebrafish larvae at 5 days post fertilization (dpf). Our high-throughput OPT system makes it possible to rapidly acquire large numbers of high-resolution 3D reconstructions and characterize the morphology of entire organs and body regions in great detail under numerous experimental conditions. Analysis of such large, dimensionally complex data sets can be facilitated by techniques developed for high-content cell-based assays: automated feature extraction and quantification, unbiased data analysis and hierarchical clustering. We have coined the term HIP to describe the application of HCS methodologies to large-scale whole-organism screens. To demonstrate the utility of HIP in zebrafish, we have performed a proof-of-concept screen focusing on the craniofacial skeleton. The head skeleton of a 5-dpf zebrafish is composed of over 30 cartilaginous elements derived from two distinct migratory cell populations—cranial neural crest and paraxial mesoderm—that are patterned by a variety of inductive signals from the surrounding tissues [11] , [12] , [13] . Because the structure and the function of the skeletal system are intimately connected, the size, shape, location and morphogenesis of all elements are tightly yet differentially regulated [12] . Genetic or teratogenic perturbations in pathways governing cell migration, proliferation or differentiation can lead to craniofacial malformations, which constitute the most common class of birth defects in humans [14] . Craniofacial anomalies (CFAs) are almost always studied in whole vertebrate models due to the strong influence of anatomical context on head skeleton morphogenesis. Even the most promising cell-based assays—such as embryoid bodies grown from embryonic stem cells—are limited to relatively simple readouts such as osteoblast formation [15] . We selected chemicals that have been functionally linked to CFAs in mammals for characterization via HIP in zebrafish (see Supplementary Table S2 ). These chemicals can be divided into three classes based on their structures and underlying mechanisms of action: (1) Retinoids (retinoic acid (RA) in the all- trans conformation (atRA), the 9 -cis isomer of RA (9 -cis -RA), the 13- cis isomer of RA (13- cis -RA) and retinol (a precursor to RA)), (2) triazole derivatives (triadimefon, fluconazole and flusilazole) and (3) steroidal alkaloids (cyclopamine). We hypothesized that malformations caused by these teratogens would differ in subtle ways that correlate with their underlying mechanism(s) of action and that such phenotypic variations would be captured by our technique and could be used to identify chemicals acting through similar mechanisms. Before CFA screening, a viability assessment was conducted by applying all chemicals at half-log intervals ranging from 3 nM to 1 mM to determine the concentration causing lethality in 50% of treated larvae (LC 50 ) under the dosing protocol ( Supplementary Table S3 ). One test chemical (Fluconazole) was eliminated from the screen because elevated mortality was not observed at the maximum screenable concentration (1 mM), and we were therefore unable to determine an LC 50 . Larvae were exposed to the chemicals starting at either 9 h post fertilization (hpf) or 30 hpf to differentiate between chemically induced effects before and after the onset of cranial neural crest migration, which begins at ~12 hpf [12] . Treatment was terminated at 3 dpf and the larvae were allowed to develop until 5 dpf. OPT imaging was carried out on fixed 5 dpf larvae stained with Alcian blue and all chemicals were assessed at the three half-log intervals immediately below the calculated LC 50 . For each larva, 320 frames were acquired at × 4 magnification with an exposure time of 0.3 ms per image frame. The acquired images where reconstructed and segmented as described above. 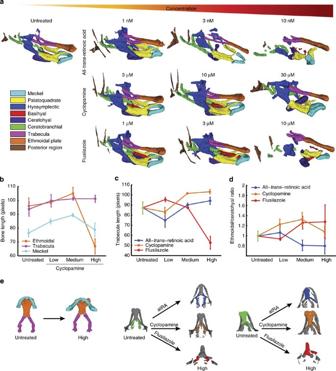Figure 2: Quantification of complex skeletal phenotypes induced by teratogenic chemicals. (a) Three-dimensional reconstructions allow visualization of complex phenotypes. Images show representative tomographic renderings of fully segmented craniofacial skeletons from 5 dpf larvae treated with three different teratogens: retinoic acid, cyclopamine and flusilazole. Representative reconstructions are shown for all chemicals at low, medium and high doses (relative to the calculated LC50) from left to right. (b) Quantitative analysis of the ethmoidal plate (orange), trabecula (pink) and Meckel’s cartilage (blue) in larvae treated with increasing concentrations of cyclopamine. Phenotypes are concentration dependent and not all bones are altered in the same manner or to the same degree. (c) Quantitative analysis of the trabeculae in larvae treated with increasing concentrations of all-trans retinoic acid (atRA; blue), cyclopamine (orange) and flusilazole (red). (d) Ratiometric analysis of the relationship between the ethmoidal plate and the ceratohyal cartilage in larvae treated with increasing concentrations of all-trans retinoic acid (atRA; blue), cyclopamine (orange) and flusilazole (red). Taken together,bthroughdshow that individual metrics reveal distinct phenotypic changes in response to different chemicals and exhibit distinct dependencies on chemical concentrations. (e) Representative reconstructions of the samples used to generate the data points inb–d. Bones colours match corresponding data points. For reconstructions ofcanddgreen bones indicate untreated (WT) controls (n=4–6 for each treatment condition,n=53 for WT,±s.e.m.). Figure 2a shows fully segmented reconstructions of representative larvae exposed to increasing concentrations of chemicals from the three different classes: atRA (a retinoid), cyclopamine (a steroidal alkaloid) and flusilazole (a triazole derivative). The progression of morphological abnormalities at increasing concentrations follows distinct patterns for each class of chemicals. For example, the angle formed between Meckel’s cartilage and the palatoquadrate is deflected ventrally by retinoids, dorsally by steroidal alkaloids, and remains unchanged by triazoles ( Fig. 2a ). Quantitative analysis of these metrics shows that individual chemicals do not alter every bone of the craniofacial skeleton in the same manner and to the same degree ( Fig. 2b ). Moreover, individual bones ( Fig. 2c ), as well as their relative lengths (ratio between two bones) ( Fig. 2d ), exhibit unique concentration-dependent responses to different chemicals (compare the trends in Fig. 2c ). This indicates that measuring the morphology of a single bone is insufficient to fully describe the phenotypic variations induced by each chemical, and measurements of multiple features and their interrelations are essential for complete characterization of phenotypes. Figure 2: Quantification of complex skeletal phenotypes induced by teratogenic chemicals. ( a ) Three-dimensional reconstructions allow visualization of complex phenotypes. Images show representative tomographic renderings of fully segmented craniofacial skeletons from 5 dpf larvae treated with three different teratogens: retinoic acid, cyclopamine and flusilazole. Representative reconstructions are shown for all chemicals at low, medium and high doses (relative to the calculated LC 50 ) from left to right. ( b ) Quantitative analysis of the ethmoidal plate (orange), trabecula (pink) and Meckel’s cartilage (blue) in larvae treated with increasing concentrations of cyclopamine. Phenotypes are concentration dependent and not all bones are altered in the same manner or to the same degree. ( c ) Quantitative analysis of the trabeculae in larvae treated with increasing concentrations of all-trans retinoic acid (atRA; blue), cyclopamine (orange) and flusilazole (red). ( d ) Ratiometric analysis of the relationship between the ethmoidal plate and the ceratohyal cartilage in larvae treated with increasing concentrations of all-trans retinoic acid (atRA; blue), cyclopamine (orange) and flusilazole (red). Taken together, b through d show that individual metrics reveal distinct phenotypic changes in response to different chemicals and exhibit distinct dependencies on chemical concentrations. ( e ) Representative reconstructions of the samples used to generate the data points in b – d . Bones colours match corresponding data points. For reconstructions of c and d green bones indicate untreated (WT) controls ( n =4–6 for each treatment condition, n =53 for WT,±s.e.m.). Full size image To quantify how much of the variation observed in individual metrics is due to actual difference in the craniofacial elements being measured and how much arises from errors in sample processing (for example, sample illumination, image processing, segmentation, and so on), we compared reconstructions obtained from (1) the same untreated control larva loaded, imaged and reconstructed multiple times, (2) multiple untreated control larvae and (3) multiple larvae exposed to 10 nM atRA ( Supplementary Fig. S4 ). Our analysis shows the variations among replicate images of the same larvae are much smaller than those among different treated and untreated larvae, indicating that the variations introduced by our imaging and image reconstruction methods are negligible. Hyperdimensional in vivo phenotyping To fully quantify the phenotypic variations in an unbiased manner, we compute a total of 202 independent metrics from each 3D reconstruction (see Supplementary Table S4 ). These metrics include lengths, 3D orientations, surface areas and volumes of different skeletal bones. To perform analyses on groups of diverse features, the metrics first need to be adjusted to a notionally common scale that also accounts for statistical variation in controls. This is done by calculating a standard score, which indicates the number of standard deviations each metric is from the mean of the control distribution and takes into account normal variation within the untreated population. This score is obtained by calculating the mean value for the metric over a large control population ( n =53), subtracting the control value from the individual metric, and dividing the difference by the standard deviation of the control population. A two-tailed Student’s t -test is also computed for each metric to calculate a P -value between the chemically treated and control larvae. These measurements are then used to construct a hyperdimensional phenotypic signature for each larva ( Fig. 3a , right panel). To determine whether the large number of metrics use in the phenotypic signature provides redundant or non-redundant information, we computed the cross-correlation between standardized metrics for all screened conditions (see Supplementary Fig. S5 ). The correlations among measured values of different metrics were low, indicating a high degree of independence across metrics (see Supplementary Fig. S3a and S3b inset). To further confirm the non-redundancy (that is, orthogonality) of our measurements, we performed principal component analysis and quantified the contribution of each metric to the overall hyperdimensional phenotypic signature. Despite the large number of metrics used, principal component analysis showed that addition of each metric contributed new and non-redundant information about the specimen (see Supplementary Fig. S3b ), indicating that HIP is more descriptive and information rich than traditional low-content phenotyping. 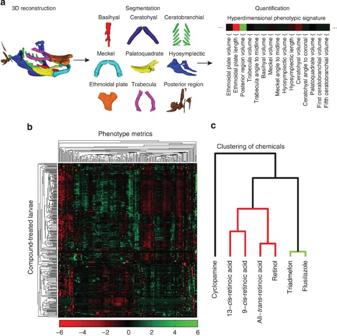Figure 3: Hyperdimensionalin vivophenotyping. (a) Schematic representation of the analysis process. Following 3D reconstruction (left) Individual bones are segmented and separated by bone type (centre). Morphological image analysis is then used to compute metrics for each bone segment (for example, volume, length, angles, surface area and location). These values are stored as a hyperdimensional phenotypic signature for each larva (right). (b) Phenotypic signature array (shown log 10 scale ofP-values). Each row represents individual larvae treated with a compound. Measurements are colour coded to indicate a reduction (red) or an increase (green) with respect to untreated controls. Phenotype metrics and compound treated larvae are ordered by hierarchical clustering based on correlation. (c) Dendrogram computed on linkage by correlation of the mean standard score for chemicals applied beginning at 9 hpf. Teratogens known to cause developmental bone abnormalities are grouped based on similarities in their hyperdimensional phenotype signature. Retinol and the retinoids (red) and the triazole derivatives (green) cluster together in groups that are distinct from cyclopamine (a steroidal alkaloid). Figure 3: Hyperdimensional in vivo phenotyping. ( a ) Schematic representation of the analysis process. Following 3D reconstruction (left) Individual bones are segmented and separated by bone type (centre). Morphological image analysis is then used to compute metrics for each bone segment (for example, volume, length, angles, surface area and location). These values are stored as a hyperdimensional phenotypic signature for each larva (right). ( b ) Phenotypic signature array (shown log 10 scale of P -values). Each row represents individual larvae treated with a compound. Measurements are colour coded to indicate a reduction (red) or an increase (green) with respect to untreated controls. Phenotype metrics and compound treated larvae are ordered by hierarchical clustering based on correlation. ( c ) Dendrogram computed on linkage by correlation of the mean standard score for chemicals applied beginning at 9 hpf. Teratogens known to cause developmental bone abnormalities are grouped based on similarities in their hyperdimensional phenotype signature. Retinol and the retinoids (red) and the triazole derivatives (green) cluster together in groups that are distinct from cyclopamine (a steroidal alkaloid). Full size image To determine whether or not hyperdimensional phenotypic signatures can reveal similarities and differences in the underlying mechanism(s) of action of test chemicals, we first performed hierarchical clustering based on the correlation of the P -values for all the samples and metrics to produce a heat map. Several distinct groups are apparent in the resultant heat map and individual larvae exposed to the same chemical at the same concentration tend to cluster together ( Fig. 3b and Supplementary Fig. S6 ). To more precisely quantify similarities and differences between chemicals, we calculated the mean standardized value for every one of the 202 metrics for each test condition (3–8 larvae per condition). Due to the extreme malformations at concentrations near the LC 50 , we eliminated the test concentration immediately below the calculated LC 50 from our analysis and included the remaining two half-log interval concentrations in our analysis. The result is a hyperdimensional phenotypic signature for each chemical that consists of 404 metrics (202 at each concentration). Cluster analysis of the hyperdimensional phenotypic signatures from our test screen produces a dendrogram with two distinct groups, one encompassing all the retinoids (red) and another emcompassing the two triazole derivatives (green; Fig. 3c ). Cyclopamine is highly uncorrelated with these two groups. Moreover, our analysis reveals similarities between retinoids and the triazole derivatives ( Fig. 3c ). These results are consistent with the known biochemical pathways and underlying mechanisms of action [16] , [17] , [18] , [19] , [20] . Vitamin A (retinol) and its active derivatives (the retinoids) regulate transcription of RA target genes and are important therapeutic agents in oncology and dermatology [18] . Triadimefon and flusilazole are triazole fungicides that act by inhibiting enzymes of the cytochrome P450 (CYP) family, including CYP26 [16] and several triazole derivatives are under investigation as CYP26-specific inhibitor [21] . CYP26 metabolizes RA to an inactive form [22] , and loss of its activity leads to increased RA-dependent gene expression and teratogenic phenotypes similar to those induced by exogenous RA in mouse and zebrafish embryos [17] , [23] . Cyclopamine, on the other hand, acts by binding to Smoothened and blocking the Hedgehog signaling pathway, which acts independently of the retinoid pathway [20] . HIP reveals additional correlations between members of the retinoid group that may reflect underlying differences in their mechanisms of action. Retinoids act primarily through two nuclear receptor families—retinoic acid receptors (RARs) and retinoid X receptors (RXRs)—which control transcription of RA target genes [18] . RARs bind both atRA and 9- cis -RA with high affinity, while RXRs preferentially bind 9- cis -RA and serve as obligatory partners for RAR and other nuclear receptors [24] . Unlike atRA and 9- cis -RA, which are biologically active ligands, retinol must first undergo enzymatic metabolism to retinaldehyde and then to RA [19] , [25] . The predominant biologically active derivative of retinol is atRA [26] . These findings agree well with our observation that the hyperdimensional phenotypic signatures of retinol and atRA cluster together on the same branch and are distinct from, but closely related to, 9- cis -RA ( Fig. 3c ). Interestingly, although 13- cis -RA shows low in vitro binding affinity to RARs and RXRs and low activity in gene expression assays [27] , [28] , it is a potent teratogen in vivo [29] and clusters with other biologically active retinoids when assessed by HIP in zebrafish larvae. HCS was developed in late 1990s to apply high-throughput techniques to the study of intact cellular systems. Over the past decade, HCS has become a mainstream technology in the pharmaceutical industry and is employed at all stages of the drug development pipeline. Increasing public availability of large-scale screening resources, through initiatives such as the Molecular Libraries Program, has also spurred an interest in HCS among academic biomedical researchers. Although HCS offers the potential to capture a vast realm of biological complexity, in practice assays are often constrained by reliance on grossly simplified biological models such as immortalized cell lines and simple culture conditions. Proposals to address these limitations typically focus on transitioning HCS assays into more biologically relevant in vitro systems such as primary cells, stem cells, 3D organotypic models and mixed co-cultures. A more powerful approach would be applying HCS directly to in vivo models that more accurately mimic normal development, disease pathology and systemic responses to perturbing agents. Here, we have demonstrated such an approach. With only minor modifications, our technology can generate high-resolution 3D reconstructions of any organ or tissue that has been labelled using a suitable chromogenic staining protocol. Of particular relevance for zebrafish researchers, our technology can easily be applied to larvae that have been stained by WISH using antisense riboprobes to visualize gene expression patterns. This can allow virtually any organ, tissue or underlying signaling pathway to be interrogated under normal and pathological conditions using HIP. When adapting OPT to new stains, it is essential to use a compatible clearing agent that optimizes the optical properties of the fixed tissue in such a way that light scattering is minimized and transmission in the visible spectra is maximized. In the case of Alcian blue, optical clearing is achieved using a 1% trypsin solution followed by equilibration in PBST. In the case of WISH, optical clearing may require imaging stained larvae in a 2:1 benzyl benzoate:benzyl alcohol solution, which is compatible with most substrates used for colorimetric detection of alkaline phosphatase activity and allows for almost complete clearing of fixed and yolk-containing tissue. By coupling high-throughput 3D tomography with automated image analysis, our platform can generate quantitative morphological metrics to create standardized phenomic databases. Phenomic databases produced by HIP can be readily compared between independent laboratories and across multiple studies. This approach allows the full diversity of morphological phenotypes in a given genetic or chemical screen to be documented and subsequently analysed using data mining and bioinformatics tools. A major strength of HIP is that it allows for unbiased screens in which mechanistic relationships can be determined without a priori knowledge. Using our platform, we are able to cluster chemicals based on their unique hyperdimensional phenotypic signatures and reveal biologically significant correlations that agree with known mechanisms of action in mammals. Importantly, at no point during this study did we need to introduce metrics that would specifically distinguish between different classes of chemicals. Automated quantitative whole-animal phenotyping technologies such as HIP will be particularly important for large-scale initiatives such as the Zebrafish Phenome Project, which aims to systematically characterize loss-of-function mutations in every protein-coding gene [30] . In addition, our technology will allow in vivo characterization of the diversity of large chemical libraries and natural-product libraries with hard-to-predict targets. Sample handling and image acquisition The system loads fixed or anaesthetized larvae from multiwell plates or reservoirs and positions them inside an ultrathin borosilicate glass capillary tube located under the field-of-view of a microscope through the use of a computerized syringe pump [9] , [10] ( Fig. 1b ). We have previously demonstrated ultrathin borosilicate glass to be an excellent capillary material due to its low autofluorescence and optical distortion [9] . A three-axis linear stage positions the loading nozzle and the computerized syringe pump aspirates the larvae into a flexible tube connected to the glass capillary. The larvae are automatically detected and positioned under the field-of-view as previously described [9] , [10] . The capillary is held by two stepper motors with hollow shafts that rotate it around its longitudinal axis. The capillary is immersed in water for refractive index matching between the inside and outside of the tube. The stepper motors rotate the capillary at a predefined speed while a high-speed camera acquires images at multiple angles. The rotation speed and timestamps assigned to each image frame are used to precisely calculate the angle of rotation of capillary at each frame. Tomographic reconstruction Before performing the tomographic reconstruction, we align the images and correct for imaging and movement artifacts. Methods describing these steps are found in the Supplementary Information . From the corrected rotational images, we reconstruct the 3D object with an iterative reconstruction method. Each of the colour channels is reconstructed independently to yield a colour 3D reconstruction. During this study we employed two different reconstruction algorithms described previously: filtered back projection (FBP) [31] and OSEM [32] . The FBP is a fast reconstruction method but does not provide the same reconstruction quality as iterative methods. Methods such as OSEM and Maximum likelihood Expectation Maximization (MLEM) [33] provide better reconstruction quality but are computationally demanding. Due to the superior speed of the FBP we use it to detect the COR, where speed is more important than the quality of reconstruction. The OSEM is an optimization of the expectation maximum reconstruction algorithm. The projection data are grouped into an ordered sequence of subsets. The iterative reconstruction is then performed on the subsets, resulting in a faster convergence. The OSEM provides significant speed increase compared with the MLEM while preserving image quality. For the whole-animal reconstruction we use OSEM method, as it provides good quality and acceptable reconstruction time. Reconstruction algorithms work under the assumption that the light rays reaching the detector undergo a rectilinear trajectory. These algorithms suffer from refraction due to index mismatch between the ultrathin capillary glass and the larva medium. As described in the Supplementary Information , we model the propagation of light through the capillary and employ the ray paths for the Radon transformation before reconstruction to compensate for this mismatch in the index refraction (see Supplementary Fig. S3 ). Image segmentation and bone identification The region(s) of interest (that is, the Alcian blue-stained cartilaginous bones of the craniofacial skeleton) were segmented from the 3D reconstruction to facilitate morphometric analyses. In general, features of interest will differ depending on the application, and there are many different 3D segmentation algorithms that can be applied to this type of data [34] . Here we used a colour-based linear discriminant analysis [35] to segment the bones from the surrounding tissue. A GUI with a slice view of the x–y , x–z and y–z planes provides the user with the ability to browse through the reconstructed sample from several angles. The user marks regions containing the desired anatomical structure (for example, Alcian blue-stained cartilage) and background regions not associated with the structure. These data serve as the training set of a classifier for identifying the desired structure. By using a linear discriminant classification, all samples in the data set can be classified according to the classes defined by the initial training set. A similar GUI isolates each segmented feature and presents it sequentially to the operator. If the segmented feature comprises a single bone, the operator can use the keypad to rapidly select the appropriate label for the bone. If the segmented feature comprises two or more bones, the operator clicks once at each side of the intersection between the bones and an algorithm automatically separates them, assigning different labels to each. If the segmented feature presented to the user is not a bone (for example, a melanophore or other high contrast structure that was mistakenly picked up by the linear discriminant classification), the user can delete the feature from the analysis. Although fully-automated algorithms can in principle be developed to segment and label the various bones of the skeleton, our semiautomated algorithm is rapid enough and sufficiently robust that a user can segment the entire skeleton accurately in less than one minute. Maintenance of fish, embryo collection and staging of larvae Zebrafish were maintained under standard laboratory conditions [36] and embryos and larvae were staged according to standard practices [37] . All procedures on live animals were approved by the Massachusetts Institute of Technology Committee on Animal Care. Cartilage staining The nomenclature for cartilaginous bones used throughout the present study is based on Kimmel et al. [37] Alcian blue staining was carried out essentially as described in previous work [13] . Briefly, at 5 dpf larvae were anaesthetized with tricaine (E10521; Sigma-Aldrich) and fixed overnight at room temperature in 10% neutral buffered formalin solution (HT5011; Sigma-Aldrich). The larvae were transferred into a solution of 0.01% Alcian blue (A5268; Sigma-Aldrich) dissolved in 80% ethanol and 20% glacial acetic acid, and stained for 20 h at room temperature. After staining, the larvae were rinsed briefly in ethanol, destained for 1 h in acidic ethanol (5% HCl, 75% EtOH, 20% H 2 O), rehydrated in PBS and the tissue was cleared in a 1% trypsin solution (T7409; Sigma-Aldrich) dissolved in 30% saturated sodium tetraborate for 6 h at room temperature. The specimens were stored in PBST at 4 °C before imaging. All Alcian blue staining steps were carried out in 24-well cell culture plates. Assay design and chemical treatment At~2–4 hpf embryos were collected and transferred into E3 medium (5 mM NaCl, 0.17 mM KCl, 0.4 mM CaCl 2 and 0.16 mM MgSO 4 ) at 28 °C. At 9 and 30 hpf, healthy embryos were arrayed into 24-well cell culture plates (four embryos per well) containing 1 ml of E3 medium. Embryos were allowed to remain in their chorions for chemical application at 9 hpf and dechorionated immediately before chemical application at 30 hpf using pronase [36] . For each treatment condition, a 100 × working stock of test chemical was prepared in 100% dimethyl sulfoxide (DMSO; for cyclopamine, 200 × working stocks were prepared in ethanol) and 10 μl of the working stock (5 μl for cyclopamine) was added to each well. Each experiment consisted of eight embryos per treatment condition (see Supplementary Table S2 ) and 53 vehicle controls (1% DMSO or 0.5% ethanol). Following treatment, embryos were continuously incubated in covered plates at 28 °C until the end of the experiment. Embryos were maintained in test chemical (without medium changes) until they reached 3 dpf, at which point they were removed from test chemical, washed briefly and raised in E3 medium until 5 dpf. Test chemicals All test chemicals were purchased from Sigma-Aldrich. CAS numbers and catalogue numbers are provided in Supplementary Table S3 . Stock solutions were prepared at 10 or 100 mM in DMSO, except for cyclopamine which was prepared as a 20 mM stock in ethanol as previously described [20] . Timings Timings were measured using the ‘clock’ functions in MATLAB and have been performed on a 96-well microtiter plate (see Supplementary Table S1 ). Times include average loading, imaging, and unloading of the samples. Other sample preparation steps (such as staining, 3D image reconstructions and image segmentation) are not included in the analysis. Statistics To calculate the P -values between the chemically treated and control larvae we employed two-tailed Student’s t -test. How to cite this article: Pardo-Martin, C. et al. High-throughput hyperdimensional vertebrate phenotyping. Nat. Commun. 4:1467 doi: 10.1038/ncomms2475 (2013).